Social evolution in structured populations Understanding the evolution of social behaviours such as altruism and spite is a long-standing problem that has generated thousands of articles and heated debates. Previous theoretical studies showed that whether altruism and spite evolve may be contingent on seemingly artificial model features, such as which rule is chosen to update the population (for example, birth–death or death–birth), and whether the benefits and costs of sociality affect fecundity or survival. Here we unify these features in a single comprehensive framework. We derive a general condition for social behaviour to be favoured over non-social behaviour, which is applicable in a large class of models for structured populations of fixed size. We recover previous results as special cases, and we are able to evaluate the relative effects of benefits and costs of social interactions on fecundity and survival. Our results highlight the crucial importance of identifying the relative scale at which competition occurs. Why would an individual help or harm others if this reduces its fitness relative to individuals that do not exhibit the social behaviour? Because such behaviours are widespread in nature, numerous theoretical studies have sought to understand the conditions for the evolution of altruism or spite. Although different theoretical frameworks and vocabularies coexist, which sometimes generated heated debates between the proponents of different schools of thought [1] , [2] , [3] , they all yield the same kind of conclusions: whether described in terms of games, or direct and indirect fitness or among and within group interactions, altruism requires some form of assortment, so that altruists interact more often with altruists than defectors do [4] , while the evolution of spite requires negative assortment [5] . Assortment occurs for instance through clustering in spatially structured (that is, ‘viscous’) populations [6] , or through conditional behaviour when there is kin or type recognition [7] , [8] , [9] . However, the conditions for the evolution of altruism or spite often depend on specific and sometimes artificial model assumptions, such as whether generations are discrete (Wright–Fisher model) or continuous (Moran [10] model) [11] , [12] . In the latter case, the sequence of events within one time step (death followed by birth, versus birth followed by death) is of crucial importance for the evolutionary outcome [13] , [14] , yet the choice itself seems arbitrary [15] . Also, in most previous models, costs and benefits of altruism or spite (that is, the ‘payoffs’) are assumed to affect the fecundity of individuals, and costs and benefits for survival have received much less attention [16] , [17] , [18] , despite the fact that such effects are equally plausible and should hence be incorporated in general models of social evolution. Here we present a comprehensive modelling framework that applies to a large class of population structures and not only unites the various assumptions in a single model, but identifies the crucial elements which support the evolution of social behaviour. In structured populations, social behaviour evolves if, for social individuals, the net social benefit of living next to other social individuals outweighs the costs of competing against them. We show that the latter depends on the way the population is updated, the type of social game that is played, and on how social interactions affect individual fecundity and survival. Dispersal and social structures of the population We consider a population of fixed size N whose structure is described by two graphs: a dispersal graph and an interaction graph , where each node, also called site, corresponds to one individual of the population. Individuals reproduce clonally, and determines dispersal patterns in the population: d ij is the fraction of the offspring produced by the individual at site i that disperse to and compete to colonize site j (∑ j d ij =1). We assume that the pattern of dispersal is similar for all individuals (technically, is transitive, see Supplementary Methods ) [14] , [18] , [19] , and is symmetrical ( d ij = d ji ), and we denote by d self = d ii the fraction of offspring that remain at their parent’s site. Most classical population structures fall into this category [19] : metapopulations, regular lattices, stepping stones, but also groups of groups, and so on (see Fig. 1 ). Social interactions are reflected in the second graph , in which e ij measures the strength of the social interaction between the individual at i and the individual at j (scaled so that ∑ i e ij =1). We denote by e self the average strength of social interactions with oneself ( e self =∑ i e ii / N ). Finally, the structural average can be interpreted as the average over all pairs of sites ( i , j ) of the chance of receiving benefits ( e ij ) from a site where offspring have been sent ( d ji ), but also as a measure of the relatedness of an individual to its social interaction partners, that is, as a measure of assortment. Hence, four parameters ( N , d self , e self , ) summarize the dispersal and social structure of the population. 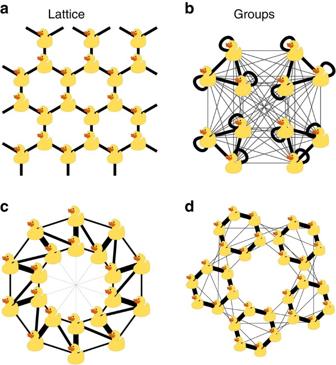Figure 1: Transitive dispersal graphs . Each duck corresponds to one individual living on one site. The thickness of a link between sitesiandjis proportional todij. (a) Lattice:dself=0;dij=1/kbetweeniand itskneighbours, anddij=0 for non neighbours; herek=3. (b) Group-structured population:dij=(1−m)/n(wheremis the chance of dispersing out of the group andnis the size of the groups; heren=3) wheniandjbelong to the same group (thick links; the loops representdself);dij=m/(N−n) wheniandjbelong to different groups (thin links). Our results are not limited to these two structures and apply to transitive graphs in general. (c) and (d) are examples of other transitive dispersal graphs . Figure 1: Transitive dispersal graphs . Each duck corresponds to one individual living on one site. The thickness of a link between sites i and j is proportional to d ij . ( a ) Lattice: d self =0; d ij =1/ k between i and its k neighbours, and d ij =0 for non neighbours; here k =3. ( b ) Group-structured population: d ij =(1− m )/ n (where m is the chance of dispersing out of the group and n is the size of the groups; here n =3) when i and j belong to the same group (thick links; the loops represent d self ); d ij = m /( N − n ) when i and j belong to different groups (thin links). Our results are not limited to these two structures and apply to transitive graphs in general. ( c ) and ( d ) are examples of other transitive dispersal graphs . Full size image A two-step life-cycle and two payoff matrices The evolution of the population is modelled using a Moran process. Each individual is either social (S) or non-social (NS). Between two time steps, exactly one individual dies and one individual reproduces, so that the size of the population remains N . The identities of the individuals who die and reproduce depend on the individuals’ fecundity and survival potential, both being affected by social interactions and by the rules according to which the population is updated. We consider two classic updating rules [13] : death–birth (DB) and birth–death (BD) (these two rules are not restricted to specific population structures, unlike some others, such as budding [20] , that are limited to deme-structured populations). In both cases, the first step (death in DB, birth in BD) involves choosing a first individual from all individuals in the population, while the second step (birth in DB, death in BD) involves only those individuals that are connected by dispersal to the site chosen in the first step (dispersal patterns being given by the graph). While previous studies only considered effects of social interactions on one of the two steps, the framework we use here allows us to consider the general case where costs and benefits of social interactions can affect both steps, that is, both fecundity and survival. Since effects on fecundity with a BD updating are equivalent to effects on survival with a DB updating in the set of population structures that we consider [19] , and vice versa , we will give all our heuristic explanations in terms of a DB updating. The fecundity and survival potential of a given individual living at site i depend on its identity (social or non-social) and on the identities of the individuals it interacts with. To which extent an individual at site j interacts with the individual at i is determined by the e ji term of the graph. The effects of this interaction on the recipient’s fecundity and survival potential are given by two general payoff matrices: In both matrices, the a (respectively b ) terms refer to payoffs received by a social individual when interacting with another social individual (respectively a non-social), and the d (respectively c ) terms refer to payoffs received by non-social individuals, when interacting with a non-social (respectively a social) individual. We use a dynamical system analysis based on moments (singlets, pairs, triplets of individuals and so on) of the distribution of social individuals in a structured population, and we assume weak selection, such that the fitness effects of interactions are small, but individuals are not necessarily phenotypically close [21] . We assume that mutations from one type to the other are rare; a new mutation only occurs after the previous one has been fixed or lost. The scales of competition The essential difference between the two steps of the process is the scale of competition (see equation (11), and Supplementary Methods ), or, using a kin selection terminology, the identity of the secondary recipients [22] at each step. In a DB updating, an increase in the survival of an individual at site i indirectly harms all the individuals who can send offspring to site i , and the magnitude of this indirect effect on j is determined by d ji . However, an increase in the fecundity of an individual i indirectly harms all other individuals j who would be competing with i for an empty site k , and the magnitude of this indirect effect on j is determined by . Hence, competition in the first step is among all individuals that are one dispersal step away, while competition in the second step is among all individuals that are two dispersal steps away. These two different competition neighbourhoods are illustrated in Supplementary Fig. 1 , in the case of a lattice-structured population. In other words, for both DB and BD updating rules, the first step, which involves choosing a first individual globally among all individuals of the population, results in a narrower competitive radius than the second step, in which another individual is chosen locally among the neighbours of the first individual [23] . Thus, whether social interactions affect the first or the second step results in a difference in the spatial scale over which social interactions affect competition. This difference turns out to be crucial for social evolution. The condition for the evolution of social behaviour We say that social behaviour evolves when the long-term frequency of social individuals is higher than the frequency of non-social individuals; or, equivalently in the limit of rare and symmetric mutations, when the probability of fixation of initially one social individual in a non-social population is higher than the converse probability of fixation: ρ S > ρ NS . Under our assumptions, we find that this condition is satisfied when This condition generalizes previous results [14] , [18] in two important ways: first, the effects of benefits and costs are not limited to fecundity but may also affect survival at the same time; second, interactions are not restricted to games with equal-gains-from-switching [24] where a − c = b − d . Equal-gains-from-switching occurs for instance in the Prisoner’s Dilemma (PD, see below) but also, to first order, in any game with small phenotypic differences between individuals [25] . With such payoffs, it is possible to find explicit expressions for ρ S and ρ NS (see Fig. 2 ). In contrast, our equation (1) also includes synergistic enhancement or discounting. 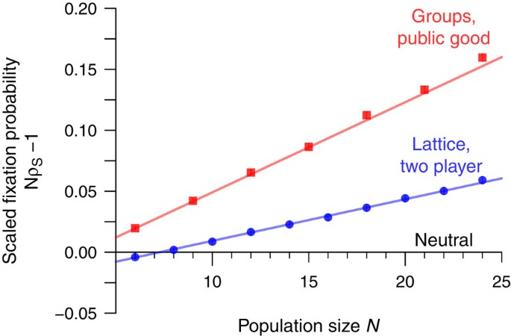Figure 2: Fixation probabilities. Comparison of the analytical fixation probabilityρSwith equal-gains-from-switching (solid coloured lines) to the frequency of fixation in numerical simulations (circles and squares), for different values of the total population sizeNand two classic population structures; results are scaled relative to 1/N, the neutral expectation. Two population structures were simulated: in blue, a lattice withk=3 neighbours, two-player games; in red, groups ofn=3 individuals with public-good games. Fixation probability: denotingB[i]=c[i]−d[i]andC[i]=d[i]−b[i], the approximate fixation probability is. Simulation data: 107runs, ±95% confidence interval (CI) (behind the dots). Parameters:b[1]=1ω,c[1]=0.1ω,b[2]=10ω,c[2]=0.5ω,ω=0.0025. Figure 2: Fixation probabilities. Comparison of the analytical fixation probability ρ S with equal-gains-from-switching (solid coloured lines) to the frequency of fixation in numerical simulations (circles and squares), for different values of the total population size N and two classic population structures; results are scaled relative to 1/ N , the neutral expectation . Two population structures were simulated: in blue, a lattice with k =3 neighbours, two-player games ; in red, groups of n =3 individuals with public-good games . Fixation probability: denoting B [ i ] = c [ i ] − d [ i ] and C [ i ] = d [ i ] − b [ i ] , the approximate fixation probability is . Simulation data: 10 7 runs, ±95% confidence interval (CI) (behind the dots). Parameters: b [1] =1 ω , c [1] =0.1 ω , b [2] =10 ω , c [2] =0.5 ω , ω =0.0025. Full size image Additional insights can be gained by defining an equivalent payoff matrix, Ã , such that condition (1) can be rewritten as (1 −1)· Ã ·(1 1) T >0. The equivalent matrix Ã can be written as For each step i of the life-cycle, σ [ i ] measures the amount of assortment due to the population structure, that is, how much individuals of the same type interact relative to individuals of different types [26] compared with how much they do in large well-mixed populations (in which σ [1] = σ [2] =1): The quantity ξ in equation (2a) measures the relative importance of the second step of the life-cycle, compared with the first: In a large well-mixed population, ξ =1. Contrasting the conditions on each step By definition of the dispersal graph , the offspring of an individual are located one dispersal step away, which happens to correspond to the competitive radius during the first step of the Moran process. Individuals are therefore directly competing against their offspring, and the detrimental effects of kin competition exactly cancel the social benefits of living next to related individuals [27] , [28] . As a result, population structure barely has any effect on the evolution of social behaviour if social interactions affect the first step of the process (see σ [1] in equation (3)), compared with large well-mixed populations. In this case, the relative effect of population structure is limited to the benefits a social individual provides to itself ( e self ), while small population sizes reduce same-type interactions: σ [1] is smaller when N is smaller. This also confirms that even with synergistic effects in the first step ( a [1] − c [1] ≠ b [1] − d [1] ), spatial structure does not facilitate the evolution of altruism [29] compared with well-mixed populations. Equation (1) also confirms that in the absence of kin discrimination or synergistic effects ( a [1] − c [1] = b [1] − d [1] ), the evolution of spite ( c [1] − d [1] <0) requires small population sizes (small N ), and limited self-interactions ( e self →0). In contrast, population structure is of crucial importance for the evolution of social behaviour whenever social interactions affect the second step of the process ( σ [2] in equation (3) and ξ in equation (4)). This is because the radius of the competitive circle is wider at the second step (two dispersal steps away): individuals are therefore competing against less related individuals, on average, than at the first step [23] . This observation had been made with specific models. For instance, conditions for general games and regular graphs of degree k (and large N ) were derived by Ohtsuki et al. [13] ; these conditions reduced to ( c [2] − d [2] )/( d [2] − b [2] )> k when a [2] − c [2] = b [2] − d [2] . For this restricted set of games, Taylor et al. [14] derived a generalization that extended to small populations sizes and covered a broad range of structures, including weighted graphs and distinct interaction and dispersal graphs. In particular, their derivation also included the ( c [2] − d [2] )/( d [2] − b [2] )> hg / l rule for regular graphs [30] , where g and h are the number of neighbours on the g and h graphs, respectively, and l the number of overlapping edges. Our formula (1) not only confirms and generalizes these findings but also offers additional insights, and we illustrate the implications of our results in Fig. 3 . 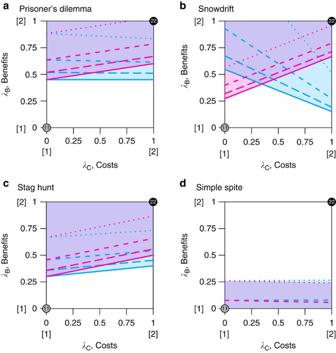Figure 3: Evolution of social behaviour under different allocations of benefits and costs. Comparing the conditions for the evolution of social behaviour (altruism in (a–c), spite in (d)), depending on whether benefits and costs affect the first or second step of the process, for four classical games. Results are shown for different population sizes (full line:N→∞, large dashed:N=60, dashed:N=24, dotted:N=12) and two structures: in magenta,dself=1/3, in cyandself=0; in both caseseself=0 and. Social individuals are favoured (ρS>ρNS) in the shaded areas. The grey (benefits and costs on the first step exclusively) and black dots (benefits and costs on the second step exclusively) in the corners correspond to the only parameter combinations that have been analysed previously in this context13,14,18,19,30. Parameters: (a) Prisoner’s dilemma,c′/b′=0.15; (b) Snowdrift,c′/(2b′−c′)=0.65; (b) Stag hunt, (b′+c′)/2b′=0.6; (d) Simple spite,c′/b′=0.02. Figure 3: Evolution of social behaviour under different allocations of benefits and costs. Comparing the conditions for the evolution of social behaviour (altruism in ( a – c ), spite in ( d )), depending on whether benefits and costs affect the first or second step of the process, for four classical games. Results are shown for different population sizes (full line: N →∞, large dashed: N =60, dashed: N =24, dotted: N =12) and two structures: in magenta, d self =1/3, in cyan d self =0; in both cases e self =0 and . Social individuals are favoured ( ρ S > ρ NS ) in the shaded areas. The grey (benefits and costs on the first step exclusively) and black dots (benefits and costs on the second step exclusively) in the corners correspond to the only parameter combinations that have been analysed previously in this context [13] , [14] , [18] , [19] , [30] . Parameters: ( a ) Prisoner’s dilemma, c ′/ b ′=0.15; ( b ) Snowdrift, c ′/(2 b ′− c ′)=0.65; ( b ) Stag hunt, ( b ′+ c ′)/2 b ′=0.6; ( d ) Simple spite, c ′/ b ′=0.02. Full size image Combining the two steps We now consider four classical games that can be expressed in terms of benefits and costs (that is, two-parameter games), and we assume that social individuals can allocate these benefits and costs in different proportions to fecundity and survival effects, or more generally to the first and second step in the life-cycle. Then the benefits and costs affecting the first step (fecundity in BD, survival in DB) are B [1] = b ′(1− λ b ) and C [1] = c ′(1− λ c ), respectively, while the benefits and costs affecting the second step (survival in BD, fecundity in DB) are B [2] = b ′(1− λ b ) and C [2] = c ′(1− λ c ), respectively. Two of the games that we consider have equal-gains-from-switching: a Prisoner's dilemma (PD) with payoff matrix on step k given by , and the equivalent spite version with negative benefits (SS), whose payoff matrices are . We also consider a Snowdrift game (SD) with payoff matrices and a Stag hunt game (SH) . For each game, we assess how the allocation of benefits and costs on either step of the life-cycle affects the evolution of social behaviour, and do so for two population structures that differ by whether an individual can be replaced by their offspring or not (that is, whether d self >0 or d self =0). The results are illustrated in Fig. 3 . We find that the optimal allocation of the benefits only depends on whether these correspond to altruism (positive benefits) or spite (negative benefits). Altruism ( Fig. 3a–c ) is most favoured if benefits are allocated to the second step of the process, which gives more weight to interactions of individuals of the same type ( σ [2] > σ [1] ). Spite, on the contrary, is more likely to evolve when the (negative) benefits affect the first step rather than the second one ( Fig. 3d ), and requires small population sizes. Let us now consider costs. In our examples, the optimal cost allocation depends on both the type of game, the size of the population ( N ) and on the fraction of an individual’s propagules that remain at the exact same site ( d self ). For example, for a sufficiently large d self (magenta lines in Fig. 3 ), altruism is most favoured if costs affect the first step of the process. With a low d self , however ( d self =0 for the cyan lines in Fig. 3 ), the allocation of the cost may not matter (for example, Fig. 3a,d , Prisoner's dilemma with large ( N ), or better be on the second step (for example, Fig. 3b , Snowdrift), or finally better be on the first step (for example, Fig. 3c , Stag hunt). While we just described cases where social interactions are of the same type on both steps, our framework also allows for the consideration of mixed cases. Focusing on games with equal-gains–from-switching, with e self =0 (like in Fig. 3a,d ), our results suggest that, behaviours that are spiteful in the first step and altruistic in the second will be favoured by selection. The simplicity and generality of our condition for the evolution of social behaviour hinges on two standard and widely used assumptions of weak selection and constant population size. Extending our results to unsaturated populations [17] , [31] , as well as to all possible network structures, is an important future challenge. Meanwhile, our results unify and generalize a great number of existing studies on the evolution of altruism or spite in structured populations, and yield new insights when social behaviour can affect both fecundity and survival. In particular, the results highlight the crucial feature determining the outcome of social evolution: the evolution of social behaviour is determined by the scale at which social interactions affect competition. Notation The population lives in an environment with N sites, labelled {1, …, N }. An indicator variable X i ( t ) gives the occupation of site i at time t : 1 (respectively 0) means that the site is occupied by a social individual (respectively non-social). Notation ‘ − ’ denotes a population average, and var S a population variance: and var S . The index S in the population variance var S is here to distinguish this variance from the variance of the state of sites ; in the same way there is a distinction between average ( − ) and expectation ( t []). We denote by the expectation of the state of the individual at site i and at time t ; a vector p ( t ) groups the expected state of all sites, and is the expected frequency of social individuals in the population at time t . Because of population structure, we also have to take into account the dynamics of pairs and triplets of individuals. We denote by the expectation of the state of pairs of sites, and group them in a matrix P ( t ). We note that the notion of relatedness classically used in kin selection studies is different and involves probabilities of identity in state or probabilities of identity by descent, without conditioning on the type of the individuals: G ij = ( X i ( t )= X j ( t )) Relatedness R ij is often defined as a standardized measure of identity [19] : where . Our measure of assortment P ij ( t ) can therefore be expressed as a function of this measure of relatedness R ij : We also need to account for associations between triplets of individuals, and we denote by the expectation of the state of triplets of sites, and group them in a three-dimensional array Π ( t ). The dispersal and social structures of the population are represented by two graphs and . We denote by d ij the fraction of the offspring of the individual living at site i that is sent to site j , and by e ij the strength of the interaction from i to j ; all these parameters are grouped in two matrices D and E . The dispersal graph is assumed to be symmetric, so that d ij = d ji (or equivalently D = D T , where T denotes transposition); the dispersal graph is also assumed to be transitive, so that the dispersal structure looks the same from every site [14] (note that the transitivity assumption is not required to derive equation (11), but it is needed to obtain explicit expressions for the expected state of pairs of individuals (equation (12))). The fecundity and survival of individuals in the population are affected by pairwise interactions with other individuals, described by the interaction graph . For our derivation, it is more convenient to rewrite the payoff matrices A [1] and A [2] (whose expressions are given in the main text) as follows: with b ′ [ i ] = c [ i ] − d [ i ] , c ′ [ i ] = d [ i ] − b [ i ] , and d ′ [ i ] = a [ i ] − b [ i ] − c [ i ] + d [ i ] . The two formulations are equivalent [32] . The effects of pairwise interactions add up, and we assume that their effects on fecundity and survival are weak, of order ω <<1: in other words, selection is weak. Note that this type of weak selection differs from weak selection due to small phenotypic differences (‘ δ -weak selection’ [21] ) classically used in kin selection models. Expected change in the frequency of social individuals We first derive a general equation for the change in the frequency of social individuals, under weak selection and for a symmetric dispersal graph ( D = D T ). We show in the Supplementary Methods how this expression relates to the Price equation [33] . Denoting by Tr( M ) the trace, that is, the sum of diagonal elements, of a matrix M , the expected change in the frequency of social individuals in the population is (details of the calculations are presented in the Supplementary Methods ): Supplementary Figure 2 (direct effects) and Supplementary Fig. 3 (secondary effects) illustrate the different terms of equation (11). The first three lines correspond to the first step (fecundity effects under BD, survival effects under DB), the last three lines to the second step (survival effects under BD, fecundity effects under DB). For each step, we can distinguish between direct effects (first column) and competition terms (second column). These competition terms correspond to secondary effects in kin selection models [22] or to circles of compensation [23] , and differ among the two steps: the competitive radius includes individuals one dispersal step away in the first step ( P · D terms), and two dispersal steps away in the second step ( P · D · D terms). This equation is dynamically not closed, because it depends on higher moments such as pairs ( P ) and triplets ( Π ) of social individuals. Evaluating the moments We show that the dynamics of pairs and triplets occur at a much faster time scale than the dynamics of the average frequency, so that we can evaluate them using a separation of time scales [34] or quasi-equilibrium approximation. Using the fact that the dispersal graph is transitive [14] , [23] and that selection is weak, we obtain the following equalities for the pairs ( 1 N , N is a N -by- N matrix containing only 1s, and I N is the identity matrix): where (details of the calculations are in the Supplementary Methods ). Note that we did not use the pair approximation [35] to derive equation (12). For triplets of individuals, we use recent results [26] , [32] showing how to express terms with triplets as functions of pairs plus a frequency-dependent term scaled by a factor α [ i ] for each step i (see Supplementary Methods for details). The α [ i ] factors will remain implicit, but they will vanish in the final condition for the evolution of social behaviour. Explicit dynamics We use the expressions we derived for pairs (equation (12)) and triplets of individuals back in the equation for the frequency dynamics (equation (11)), thus arriving at a closed dynamical system, given below in equation (16). We denote by d self = d ii , the fraction of propagules that remain at their parent's site (the same for all sites i on a transitive graph), by the average interaction with oneself, and finally a compound parameter summarizing the dispersal and interaction graphs (recall that d kl = d lk ), that can be interpreted as the average chance of receiving benefits ( e lk ) from a site where offspring have been sent ( d kl ). We then define two compound parameters, σ and τ , that depend on the population structure and the different payoffs: and With these definitions, we find that the expected change in the frequency of social individuals can be written as follows: In other words, the structured population behaves as a well-mixed one, under linear frequency-dependent selection given by s ( p ( t )). Fixation probabilities The fixation probability of a single mutant under a Moran process with a linear frequency-dependent selection coefficient is a classical result [36] , [37] , [38] . Accordingly, the fixation probability of a social mutant in a population of non-social individuals, when selection is weak, can be approximated as Reciprocally, the fixation probability of initially one non-social individual in a population of social individuals is We define the evolutionary success of social individuals by the condition Using equations (17) and (18), this condition becomes . Finally, using the definitions (14) and (15) we obtain equation (1) in the main text. Simulations Stochastic simulations were coded in C; the population was updated following a Moran process as described in the main text, and the simulation stopped when the social trait was either fixed or lost. Fixation probabilities, with initially only one social individual in the population, were estimated after 10 7 runs for each parameter combination. The simulation scripts are available on Dryad: doi:10.5061/dryad.r28qk . How to cite this article : Débarre, F. et al. Social evolution in structured populations. Nat. Commun. 5:3409 doi: 10.1038/ncomms4409 (2014).